Freely orbiting magnetic tweezers to directly monitor changes in the twist of nucleic acids The double-stranded nature of DNA links its replication, transcription and repair to rotational motion and torsional strain. Magnetic tweezers (MT) are a powerful single-molecule technique to apply both forces and torques to individual DNA or RNA molecules. However, conventional MT do not track rotational motion directly and constrain the free rotation of the nucleic acid tether. Here we present freely orbiting MT (FOMT) that allow the measurement of equilibrium fluctuations and changes in the twist of tethered nucleic acid molecules. Using a precisely aligned vertically oriented magnetic field, FOMT enable tracking of the rotation angle from straight forward ( x,y )-position tracking and permits the application of calibrated stretching forces, without biasing the tether's free rotation. We utilize FOMT to measure the force-dependent torsional stiffness of DNA from equilibrium rotational fluctuations and to follow the assembly of recombination protein A filaments on DNA. The degree of twist of the intertwined strands that form the DNA duplex is altered by numerous cellular processes, including replication, transcription, repair and the binding of small molecules or proteins to DNA. Magnetic tweezers (MT; Supplementary Fig. S1 ) are a powerful technique to report on such processes, as they permit the application of forces and torques to single nucleic acid molecules tethered between a surface and micron-sized magnetic particles [1] , [2] , [3] , [4] . However, conventional MT do not track rotational motion directly, and both MT and the recently developed magnetic torque tweezers (MTT) [5] , [6] , [7] constrain the free rotation of the magnetic particles. Here we present a new implementation of MT, termed freely orbiting MT (FOMT) that enables simple, direct and unbiased measurement of changes in the twist of the tether. The measurement relies on carefully aligning a cylindrical magnet above the sample, such that the magnetic field lines are predominantly vertically aligned with the DNA tether axis. We demonstrate that for this magnet geometry, the tethered bead undergoes Brownian fluctuations in x and y that lies on a perfectly circular annulus. The ( x,y ) fluctuations are tightly coupled to the rotation of the bead around its axis: the same face of the bead always points toward the centre of the circular annulus, similar to the rotation of the moon around the earth. This one-to-one coupling between the bead's ( x,y ) position and its angular orientation allows us to measure the rotation angle and to track changes in the twist of the DNA tether, solely by tracking the bead's spatial ( x,y ) coordinates, entirely obviating the need for any special angular tracking protocols. Importantly, we demonstrate that in our FOMT configuration, the bead's rotation about the tether axis is essentially unconstrained by the magnets, that is, the magnetic field contributes much less than the thermal energy k B T to the energy barrier for full-bead rotation, and the bead's rotation is solely constrained by the tether. We present applications of the FOMT technique to measurements of the force-dependent torsional stiffness of DNA from equilibrium fluctuations and to the real-time observation of the changes in linking number that accompany the assembly of recombination protein A (RecA) heteroduplex filaments. Finally, we compare and contrast the FOMT method with a number of alternative single-molecule approaches to measuring nucleic acid twist. Forces and torques in MTs At the heart of FOMT are superparamagnetic beads tethered to a flow cell surface via double-stranded DNA (dsDNA) tethers ( Fig. 1a ). We use a cylindrical magnet mounted on a motor-controlled vertical linear stage above the surface to apply upward forces to the magnetic beads that stretch the DNA tether. The force exerted on the magnetic beads by the external magnetic field B depends on their total magnetization m(B) and is proportional to the gradient of the magnetic field [8] . In contrast, the torque applied to the beads by the magnetic field depends on the preferred magnetization axis, m 0 , and is given by [3] : Γ B =m 0 × B . If B is aligned vertically as in FOMT, m 0 aligns vertically and the torque from the magnet about the z axis, equal to m 0,x B y (or m 0,y B x ), is negligible. In contrast, the magnetic fields in conventional MT and MTT have large enough horizontal components to constrain the beads' rotation about the z axis, as a result of which the beads will faithfully follow rotation of the permanent magnets [3] , [6] . 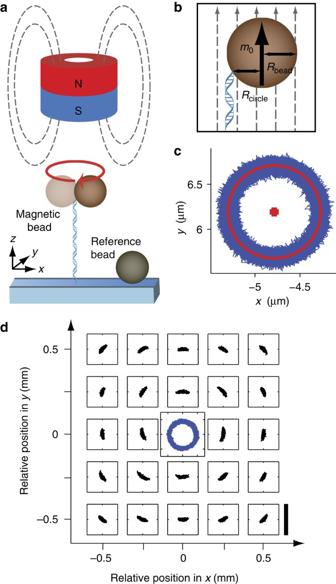Figure 1: Schematic of FOMT. (a) In the FOMT, a superparamagnetic bead is tethered to a flow cell surface via a dsDNA construct with multiple attachment points at both ends. A cylindrical magnet exerts a magnetic field that is predominantly aligned in thezdirection. A reference bead is attached to the flow cell surface and tracked simultaneously to correct for mechanical drift. (b) The preferred magnetization axism0of the bead aligns with the field along thezaxis. In this geometry, the bead can freely rotate about thezaxis, tracing out a circle of radiusRcircle. (c) (x,y) Fluctuations of a bead tethered to a 7.9 kb DNA under a well-aligned cylindrical magnet with a fitted circle. (d) (x,y) Fluctuations of the bead as a function of magnet position. The position of the cylindrical magnet was scanned at a constant height of 3 mm across the flow cell surface in steps of 250 μm inxandy. Position of the bead relative to the magnet is indicated on the outer plot axes. At each magnet position, fluctuations of the same DNA-tethered bead were recorded and are plotted in the small square coordinate systems (scale bar is 2 μm). A systematic variation of the (x,y)-fluctuation pattern with magnet position resembling a cyclone or vortex is apparent. For a well-centered magnet, the bead's (x,y) fluctuations trace out a circular trajectory, plotted in the centre of the plot. This trace was recorded in a separate experiment after aligning the magnets in smaller steps about the centre and is shown for illustration in this plot. Figure 1: Schematic of FOMT. ( a ) In the FOMT, a superparamagnetic bead is tethered to a flow cell surface via a dsDNA construct with multiple attachment points at both ends. A cylindrical magnet exerts a magnetic field that is predominantly aligned in the z direction. A reference bead is attached to the flow cell surface and tracked simultaneously to correct for mechanical drift. ( b ) The preferred magnetization axis m 0 of the bead aligns with the field along the z axis. In this geometry, the bead can freely rotate about the z axis, tracing out a circle of radius R circle . ( c ) ( x,y ) Fluctuations of a bead tethered to a 7.9 kb DNA under a well-aligned cylindrical magnet with a fitted circle. ( d ) ( x,y ) Fluctuations of the bead as a function of magnet position. The position of the cylindrical magnet was scanned at a constant height of 3 mm across the flow cell surface in steps of 250 μm in x and y . Position of the bead relative to the magnet is indicated on the outer plot axes. At each magnet position, fluctuations of the same DNA-tethered bead were recorded and are plotted in the small square coordinate systems (scale bar is 2 μm). A systematic variation of the ( x,y )-fluctuation pattern with magnet position resembling a cyclone or vortex is apparent. For a well-centered magnet, the bead's ( x,y ) fluctuations trace out a circular trajectory, plotted in the centre of the plot. This trace was recorded in a separate experiment after aligning the magnets in smaller steps about the centre and is shown for illustration in this plot. Full size image Bead fluctuations in the FOMT lie on a circular annulus The excursions in ( x,y ) of a magnetic bead tethered by a single dsDNA tether depend strongly on the position of the tether with respect to the axis of the cylindrical magnet ( Fig. 1 ; Supplementary Figs S2–S3 ). When the magnet is far from being centered on the tethered bead, the fluctuations in x and y are uncoupled and Gaussian distributed, similar to the fluctuations observed in conventional MTs ( Supplementary Figs S2–S4 ). As the cylindrical magnet is progressively centered on the magnetic bead, the ( x,y ) fluctuations become coupled and trace out circular arcs. If the cylindrical magnet is centered on the bead to within ∼ 10 μm, the torque from the magnets about the z axis is reduced to the point that thermal fluctuations suffice to rotate the bead around its attachment point. Consequently, the fluctuations in ( x,y ) are strongly coupled and trace out a circular annulus with radius R circle , where R circle is the radial distance between the DNA attachment point and the bead's centre ( Fig. 1b,c ). The overall fluctuation pattern resembles a cyclone or vortex ( Fig. 1d ; Supplementary Figs S2 and S3 ) and provides a straightforward operational way to centre the alignment of the magnet by iteratively moving the magnet towards the middle of the arc. We observe similar, cyclone-like patterns for DNA constructs of different length and beads of different sizes ( Supplementary Figs S2 and S3 ). The fluctuation pattern under the cylindrical magnet is a consequence of the vertically aligned field and not of the circular symmetry of the magnet, as evidenced by the fact that a pair of magnets aligned in a vertical–parallel configuration yields a very similar pattern of fluctuations ( Supplementary Fig. S5 ). In contrast, the ( x,y ) fluctuations in conventional MT do not show significant variation with the scanned magnet position ( Supplementary Fig. S4 ). A number of predictions about the size of R circle from simple geometric considerations ( Fig. 1b ) are borne out experimentally. First, R circle lies between zero (for a bead tethered at the south pole) and ≈ R bead (for a bead tethered at or above the equator). Experimentally, we indeed consistently find 0≤ R circle ≤ R bead + L P , where L P ≈50 nm is the persistence length of DNA, which is unsurprising when one considers that the DNA may protrude from the equator by up to ≈ L P ( Supplementary Fig. S6 ; Supplementary Table S1 ). Second, flipping the magnet (that is, north up versus north down) systematically affects both circle radius R circle and the apparent tether length 〈 z 〉 ( Supplementary Fig. S6 ; Supplementary Table S1 ). The correlated changes in R circle and 〈 z 〉 can be understood from a geometric argument as follows. We begin by considering a bead tethered in its lower hemisphere ( Supplementary Fig. S6a , left), such that it rotates directly about the tether attachment point. The radius of the circle is a measure of the 'latitude' of tether attachment φ =arcsin( R circle,lower /R bead ). To understand the height of the bead above the surface, 〈 z 〉, from the stretched extension of the DNA tether, L , we first note that 〈 z 〉= L holds true only if the bead is tethered at the south pole. For a bead tethered anywhere in the lower hemisphere, 〈 z 〉 lower = L−R bead (1−cos(φ)), where the second term is the length correction d , also used in the calibration of the forces; see below. When the magnet is flipped, the bead rotates by 180° in the plane of the page, as a result of which the tether attachment point moves to the upper hemisphere ( Supplementary Fig. S6a , right). In this new situation, the radius of the circle is maximal and equals approximately R circle,upper ≈ R bead . In practice, we find R circle,upper ≈ R bead + L P where L P is the persistence length of DNA, indicating that the DNA protrudes from the surface by ≈ L P . For a bead tethered in the northern hemisphere, the DNA tether wraps around the upper surface of the bead and extends down from the equator, such that 〈 z 〉 upper = L – R bead (1+π/2−φ). Combining the considerations for the two tether geometries, we predicted the change in bead height upon flipping the magnet to equal Δ z =〈 z 〉 lower −〈 z 〉 upper = R bead (cos(φ)+π/2−φ). The experimentally observed changes in 〈 z 〉 agree with the predicted values for z within 20% ( Supplementary Table S1 ). The predicted Δ z tends to somewhat smaller than the observed values, which would be expected if the DNA tether does not follow the surface of the bead closely in the northern hemisphere, but undergoes excursions on the length scale of L P . Third, R circle is approximately independent of the stretching force ( Fig. 2 ; Supplementary Fig. S7 ). Fourth, the height of the bead above the surface 〈 z 〉 varies systematically with the global alignment of the magnet ( Supplementary Fig. S8 ). 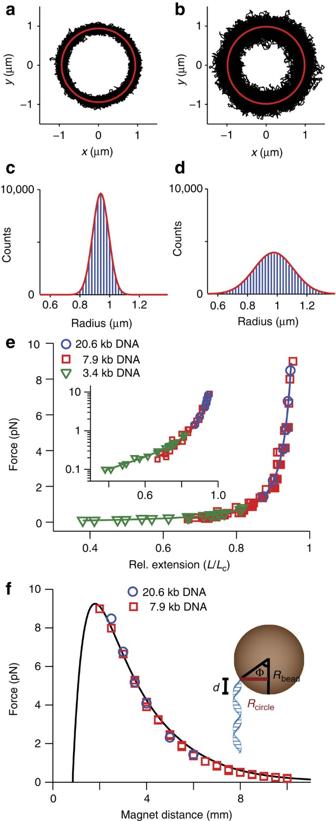Figure 2: Force calibration and force-extension measurements in the FOMT. (a) (x,y) Fluctuations (black) of a bead tethered by a 20.6-kb DNA construct under the cylindrical magnet with the magnet at a distance of 2 mm from the flow cell surface, corresponding to a high stretching force (8.5 pN). The fluctuations lie on a circular annulus (red line). (b) (x,y) Fluctuations (black) and fitted circle (red) for the same tethered bead as in (a) with the magnet at a distance of 6 mm from the flow cell surface, corresponding to a lower stretching force (1.5 pN). (c) Histogram of the fluctuations in the radial coordinate for the data from (a). The red line is a Gaussian fit with s.d. ofσ=0.0542 μm. (d) Histogram of the fluctuations in the radial coordinate for the data from (b). The red line is a Gaussian fit with s.d. ofσ=0.133 μm. (e) Force-extension data for DNA tethers of different length stretched using the cylindrical magnet geometry. Forces and DNA extensions were calibrated as described in the main text. Data are for 3.4 kb DNA using 0.5 μm diameter MagSense beads, and for 7.9 and 20.6 kb DNA using M270 beads. Extensions were scaled by the contour length to facilitate the comparison of the different length molecules. The lines are fits of the WLC model10. The inset shows the same data with a logarithmically scaled force axis. (f) Stretching forces for M270 beads as a function of distance of the cylindrical magnet from the flow cell surface. The flow cell used in these experiments has a thickness of ≈400 μm. Experimental data for 7.9 kb tethers and 20.6 kb tethers. The black line is a prediction from first principle calculations taking into account the magnetic field and the beads' magnetization (Supplementary Figs S11andS12). The inset shows the bead and tether geometry used for force and length determination. Figure 2: Force calibration and force-extension measurements in the FOMT. ( a ) ( x,y ) Fluctuations (black) of a bead tethered by a 20.6-kb DNA construct under the cylindrical magnet with the magnet at a distance of 2 mm from the flow cell surface, corresponding to a high stretching force (8.5 pN). The fluctuations lie on a circular annulus (red line). ( b ) ( x,y ) Fluctuations (black) and fitted circle (red) for the same tethered bead as in ( a ) with the magnet at a distance of 6 mm from the flow cell surface, corresponding to a lower stretching force (1.5 pN). ( c ) Histogram of the fluctuations in the radial coordinate for the data from ( a ). The red line is a Gaussian fit with s.d. of σ =0.0542 μm. ( d ) Histogram of the fluctuations in the radial coordinate for the data from ( b ). The red line is a Gaussian fit with s.d. of σ =0.133 μm. ( e ) Force-extension data for DNA tethers of different length stretched using the cylindrical magnet geometry. Forces and DNA extensions were calibrated as described in the main text. Data are for 3.4 kb DNA using 0.5 μm diameter MagSense beads, and for 7.9 and 20.6 kb DNA using M270 beads. Extensions were scaled by the contour length to facilitate the comparison of the different length molecules. The lines are fits of the WLC model [10] . The inset shows the same data with a logarithmically scaled force axis. ( f ) Stretching forces for M270 beads as a function of distance of the cylindrical magnet from the flow cell surface. The flow cell used in these experiments has a thickness of ≈400 μm. Experimental data for 7.9 kb tethers and 20.6 kb tethers. The black line is a prediction from first principle calculations taking into account the magnetic field and the beads' magnetization ( Supplementary Figs S11 and S12 ). The inset shows the bead and tether geometry used for force and length determination. Full size image Tracking of rotation angle from ( x,y ) position Under the well-aligned cylindrical magnet, rotation about the DNA tether is tightly coupled to motion on the circular annulus and the rotation angle can be determined by converting the ( x,y ) position to polar ( r,θ ) coordinates (Methods; Supplementary Figs S9 and S10 ). The rotation angle determined from the ( x,y ) position is in excellent agreement with the results of direct tracking of the bead's rotation [6] , based on image analysis of magnetic beads with small non-magnetic fiducial marker beads attached ( Supplementary Figs S9 and S10 ). The FOMT geometry, therefore, enables precise measurement of tether rotation from simple ( x,y )-position tracking, without the need for fiducial markers or a designated angular tracking protocol. Force calibration from analysis of the radial fluctuations The stretching force F exerted in the FOMT can be accurately calibrated from analysis of the thermal fluctuations in the radial coordinate r by adapting the approach used for conventional MTs [1] , [3] , [8] ( Fig. 2 ; Supplementary Figs S11 and S12 ). The radial fluctuations deduced from the ( x,y ) position on the circular annulus are Gaussian, with a standard deviation that depends on the vertical distance between the magnet and the flow cell ( Fig. 2a–d ). Using the equipartition theorem, the stretching force exerted by the cylindrical magnet can be determined [1] , [4] , [9] from the variance of the radial fluctuations 〈 (r–r 0 ) 2 〉: where rθ 0 is the mean radius and the angled brackets denote the time average. The tether length L is given by L =〈 z 〉 +d , where the length correction d is given by d = R bead (1−cos(φ)) with sin(φ)= R circle / R bead ( Fig. 2f , inset). In practice, it is advantageous to carry out the force calibration in Fourier space by considering the power spectrum of the radial fluctuations to which corrections for camera blurring and aliasing can be applied, again in exact analogy to the analysis of the x or y fluctuations in conventional MT [9] . Using this analysis, we determined the force-extension response of dsDNA under the well-aligned cylindrical magnet for 3.4, 7.9 and 20.6 kb DNA constructs, respectively. The data are well described by the worm-like chain model of entropic DNA elasticity [10] ( Fig. 2e ), with fitted values for the persistence length of L P ≈45 nm and values for the contour length of L C =1.1±0.1, 2.75±0.1 and 7.1±0.2 μm for the different length DNA constructs, respectively, in good agreement with the values expected from the crystallographic length of DNA. In addition, we find excellent agreement between the forces determined from the analysis of the thermal fluctuations in the radial coordinate and predictions of the forces from first principles [8] ( Fig. 2f ; Supplementary Figs S11 and S12 ). Rotational fluctuations in the FOMT We demonstrate that in the FOMT geometry, the bead's rotational fluctuations about the tether axis are constrained only by the torsional stiffness of the dsDNA tether and not by the magnet. The bead position in the ( x,y ) plane exhibits a nearly uniform distribution around the circular annulus ( Fig. 3a ), suggesting that there are no preferred positions induced by the magnets. The corresponding time trace θ ( t ) of angular fluctuations (obtained from conversion of the ( x,y ) positions) reveals large excursions corresponding to several full turns ( Fig. 3b ). The distribution of angular fluctuations, P ( θ ), is Gaussian with a width of σ θ =223° ( Fig. 3c ). The energy landscape implied by the rotational fluctuations, U ( θ )=− k B T ln( P ( θ )), is well described by the harmonic approximation, U harm ( θ )=−( k θ /2)( θ–θ 0 ) 2 ( Fig. 3d ). The torsional spring constant is given by the equipartition theorem: The fact that the deviations from the harmonic approximation are much smaller than k B T over a range of >1,000° and show no periodicity corresponding to 360° ( Fig. 3d ) indicates that the influence of the magnets on the rotational motion is negligible, as any biasing potential exerted by the magnets would have a periodicity of 360° or less. The absence of any periodic preferred positions induced by the magnets is further supported by the absence of any peaks or features in the pairwise autocorrelation of the angle and its Fourier transform ( Supplementary Fig. S13 ). Furthermore, if the tether loses its torsional constraint, angular fluctuations of even larger amplitude are observed, consistent with purely diffusive motion in the angular coordinate ( Supplementary Fig. S14 ). The characteristic time scale τ c of fluctuations in the harmonic potential is given by τ c =γ/k θ , where γ is the friction coefficient of the tethered bead. We find good agreement between τ c , determined from analysis of the temporal autocorrelation or the power spectrum of the angular fluctuations ( Fig. 4e,f ), and predictions from the bead geometry (Methods). 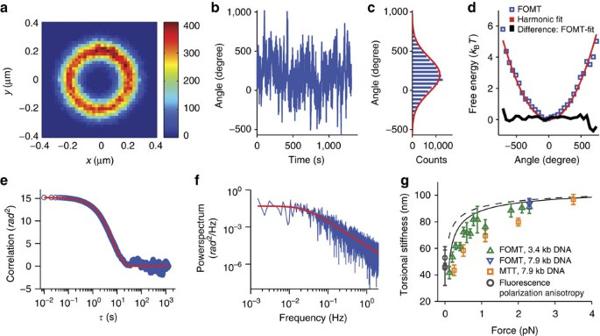Figure 3: Rotational fluctuations in the FOMT are constrained by the torsional stiffness of DNA only. Data in panelsa–fwere obtained using a 0.35μm radius bead and a 3.4-kb dsDNA tether in the FOMT geometry. (a) Histogram of the (x,y) fluctuations (seeSupplementary Fig. S13for additional plots of the same trace). The histogram reveals essentially uniform coverage of the positions on the circle. (b) Rotational fluctuations of the bead determined from the (x,y) positions. (c) Histogram of the rotational fluctuations. The red line is a Gaussian fit withσθ=223°. (d) The energy landscape implied by the rotational fluctuation density from (b). The difference between the landscape implied by the rotational fluctuations and the harmonic approximation (withkθ=kBT/σθ2=0.27 pN.nm/rad) is much smaller than the thermal energykBT. Data are offset for clarity such thatθ0=0. (e) Temporal autocorrelation of the rotational fluctuations. The red line is an exponential fit with the trap stiffnesskθ=0.27 pN.nm/rad and the friction coefficientγ=1.82 pN.nm.s implying a characteristic timeτc=γ/kθ=6.75 s. (f) Power spectrum of the rotational fluctuations. The red line is a Lorentzian fit with the corner frequencyfc=0.024 Hz, in excellent agreement with the value expected from the temporal autocorrelation using the relationshipfc=1/(2πτc). (g) Effective DNA torsional stiffness as a function of applied stretching force determined from equilibrium fluctuations (equation 4). Data are the mean and s.e.m. from at least five independent measurements in PBS+ buffer. MTT6and fluorescence polarization anisotropy11,12,13data are shown for comparison. Predictions from the first- and third-order Moroz–Nelson model are shown as dashed and solid lines, respectively. Figure 3: Rotational fluctuations in the FOMT are constrained by the torsional stiffness of DNA only. Data in panels a–f were obtained using a 0.35μm radius bead and a 3.4-kb dsDNA tether in the FOMT geometry. ( a ) Histogram of the ( x,y ) fluctuations (see Supplementary Fig. S13 for additional plots of the same trace). The histogram reveals essentially uniform coverage of the positions on the circle. ( b ) Rotational fluctuations of the bead determined from the ( x,y ) positions. ( c ) Histogram of the rotational fluctuations. The red line is a Gaussian fit with σ θ =223°. ( d ) The energy landscape implied by the rotational fluctuation density from ( b ). The difference between the landscape implied by the rotational fluctuations and the harmonic approximation (with k θ = k B T / σ θ 2 =0.27 pN.nm/rad) is much smaller than the thermal energy k B T . Data are offset for clarity such that θ 0 =0. ( e ) Temporal autocorrelation of the rotational fluctuations. The red line is an exponential fit with the trap stiffness k θ =0.27 pN.nm/rad and the friction coefficient γ =1.82 pN.nm.s implying a characteristic time τ c = γ/k θ =6.75 s. ( f ) Power spectrum of the rotational fluctuations. The red line is a Lorentzian fit with the corner frequency f c =0.024 Hz, in excellent agreement with the value expected from the temporal autocorrelation using the relationship f c =1/(2π τ c ). ( g ) Effective DNA torsional stiffness as a function of applied stretching force determined from equilibrium fluctuations (equation 4). Data are the mean and s.e.m. from at least five independent measurements in PBS+ buffer. MTT [6] and fluorescence polarization anisotropy [11] , [12] , [13] data are shown for comparison. Predictions from the first- and third-order Moroz–Nelson model are shown as dashed and solid lines, respectively. 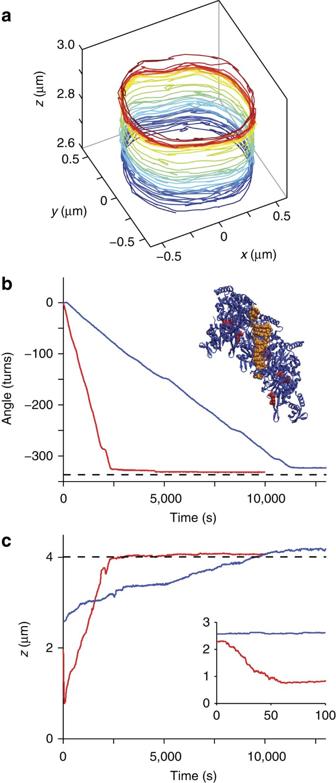Figure 4: RecA filament formation on dsDNA monitored in the FOMT. Assembly of RecA heteroduplex filaments on 7.9 kb DNA in the presence of ATP-γS. (a) (x,y,z) Trajectory during the first 1,000 s of filament assembly (Rbead=1.4 μm,F=6.5 pN). Colour indicates time from blue to red. The bead traces out a spiral as RecA assembly unwinds and lengthens the DNA. (b) Rotation angle as a function of time during RecA assembly for (Rbead=1.4 μm,F=6.5 pN; blue) and for (Rbead=0.5 μm,F=1.5 pN; red). The inset shows the crystallographic structure20of RecA (blue) bound to DNA (orange) exhibiting a binding stoichiometry of one RecA monomer per 3 bp DNA (PDB accession code 3CMT). ATP analogues bound at the RecA monomer interfaces are shown in red. (c) Time traces of the bead heightz(same colour code as b). The inset shows the first 100 s. The bead atF=1.5 pN initially moves down because of DNA supercoiling. The predictions from the crystallographic structure20are shown as dashed lines in (b) and (c). Full size image Figure 4: RecA filament formation on dsDNA monitored in the FOMT. Assembly of RecA heteroduplex filaments on 7.9 kb DNA in the presence of ATP-γS. ( a ) ( x,y,z ) Trajectory during the first 1,000 s of filament assembly ( R bead =1.4 μm, F =6.5 pN). Colour indicates time from blue to red. The bead traces out a spiral as RecA assembly unwinds and lengthens the DNA. ( b ) Rotation angle as a function of time during RecA assembly for ( R bead =1.4 μm, F =6.5 pN; blue) and for ( R bead =0.5 μm, F =1.5 pN; red). The inset shows the crystallographic structure [20] of RecA (blue) bound to DNA (orange) exhibiting a binding stoichiometry of one RecA monomer per 3 bp DNA (PDB accession code 3CMT). ATP analogues bound at the RecA monomer interfaces are shown in red. ( c ) Time traces of the bead height z (same colour code as b). The inset shows the first 100 s. The bead at F =1.5 pN initially moves down because of DNA supercoiling. The predictions from the crystallographic structure [20] are shown as dashed lines in ( b ) and ( c ). Full size image DNA torsional stiffness from angle fluctuations In the absence of any torsional constraint by the magnets in the FOMT, the free rotation of the bead is limited only by the dsDNA tether. The stiffness of the torsional trap imposed by the dsDNA tether is given by where C and L C are the effective torsional persistence length and contour length of DNA, respectively. We can relate the width of the rotational fluctuations σ θ directly to the effective torsional stiffness C by combining equations (2) and (3): Using equation (4), we have measured C for fully dsDNA tethers and find a substantial dependence on stretching force ( Fig. 3 g ): C increases from 42±6 nm at F =0.1 pN to larger values at higher forces. Our results at low forces agree, within experimental error, with previous fluorescence polarization anisotropy measurements made on short, linear DNA constructs that are effectively at zero stretching force [11] , [12] , [13] . In addition, the FOMT results agree, within experimental error, with MTT measurements [6] , and give similar results for 3.4 and 7.9 kb DNA ( Fig. 3g ). Moroz–Nelson model for DNA torsional stiffness We compare the experimental measurements of the effective torsional stiffness C of DNA with the model derived by Moroz and Nelson [14] , [15] ( Fig. 3g ). The model uses a perturbative approach with an expansion valid for large forces. Frequently, the approximate result to first order, ∼ O( F − 1/2 ), has been used in both theoretical analyses [16] and in the interpretation of experimental results [6] , [17] . Here, we compare the first-order results with the more accurate third-order approximation, ∼ O( F − 3/2 ) (ref. 18 ): where C lim =109 nm is the (intrinsic as opposed to effective) torsional stiffness of DNA [15] and L P is the bending persistence length ( L P =43±3 nm; Supplementary Fig. S11d ). The value of C lim =109 nm is in good agreement with the data at high force measured independently with a rotary bead assay [19] and with MTT [6] , under similar buffer conditions. Although both the first- and third-order approximations overestimate the experimentally measured values for C(F) at low F , the third-order approximation provides a better description of the experimental data (reduced χ 2 =5.7 and 16.25, for the third- and first-order models, respectively). Alternatively, the intrinsic torsional stiffness of DNA C lim can be treated as a free parameter and fits to the FOMT data. In this case, the best fit for the third-order approximation is obtained with C lim =95 nm (reduced χ 2 =2.0) and for the first-order approximation with C lim =88 nm (reduced χ 2 =5.7). Treating C lim as a free parameter improves the fit at low forces, but leads to poorer agreement at high forces, as is to be expected. Monitoring RecA filament formation in the FOMT We demonstrate the capability of FOMT to monitor dynamical changes in the twist of DNA tethers by monitoring the assembly of RecA filaments on DNA. Upon addition of RecA and the non-hydrolyzable ATP-analog ATP- γ S, beads held in the FOMT, trace out spiralling trajectories, indicating that the DNA tethers lengthen while being unwound ( Fig. 4a ). We can follow the assembly of the heteroduplex filament to completion by monitoring θ ( t ) and z ( t ) over thousands of seconds ( Fig. 4b,c ; Supplementary Table S2 ), and observe a total unwinding of the 7.9 kb DNA to −328±10 turns and a lengthening to 4.1±0.1 μm. Given the binding stoichiometry of one RecA monomer per three DNA base pairs, our measurements imply a overall change in twist of −44.7±1.4° and a length change of 0.53±0.04 nm per RecA monomer, in good agreement with the −45.8° twist and 0.49 nm length changes per RecA determined from crystallography [20] . In addition to revealing the overall filament structure, the FOMT measurements provide insights into the dynamics of the assembly process. To demonstrate this, we consider in detail the RecA assembly traces at a stretching force of F= 1.5 pN ( Fig. 4c , red curve; Supplementary Fig. S15 ). Although the rotation rate is nearly constant throughout the reaction, the behaviour of the apparent tether length reveals two phases: first, a rapid decrease (up to ∼ 75 s as shown in red curve in inset to Fig. 4c ; see also inset to Supplementary Fig. S15 ) and subsequently, a slow increase ( Fig. 4c , red curve). The initial decrease in the tether extension is consistent with plectoneme formation. After all, if RecA polymerization and its concomitant DNA unwinding occurs considerably more rapidly than the bead can relax in the angular coordinate because of its torsional drag, compensatory changes in twist or writhe must be introduced to preserve the linking number. Initially these take the form of changes of the twist, ΔTw , of the DNA tether, leading to the accumulation of torsional strain. However, once the buckling torque is reached, additional RecA assembly is compensated by changes in writhe, ΔWr , that is, the formation of plectonemic supercoils. We can estimate the torque in the tether during this initial phase from the bead rotation rate d θ/ d t ( Fig. 4b , red curve): Γ DNA = Γ drag = γ ·d θ/ d t . We find Γ DNA ≈10 pN nm −1 and 14 pN nm −1 for tethers attached to 0.5 and 1.4 μm radius beads, respectively ( Fig. 4b,c ; Supplementary Fig. S15 ), which agree well with previous measurements of DNA buckling torque at this stretching force [6] , ≈14 pN nm −1 , consistent with the formation of plectonemes during the initial phase of RecA filament assembly. By considering both the rate of bead rotation d θ/ d t and the rate of change of the apparent tether length d z/ d t during the initial assembly phase, we can also compute the RecA assembly rate, d N RecA /d t , during plectoneme formation at the buckling torque. The rate of bead rotation equals where Δθ RecA is the change in DNA twist induced by binding a single RecA monomer and d Wr/ d t and d Tw/ d t are the rate of change of writhe and twist, respectively. If the molecule is already at the buckling torque, d Tw/ d t= 0. The rate of plectoneme formation, d Wr/ d t, can be deduced from the change in the apparent tether length where Δl RecA is the length increase due to binding of a single RecA monomer to duplex DNA, and Δl plec is the contour length of DNA stored within a single plectoneme. Combining equations (6) and (7) to eliminate d Wr /d t , we obtain an expression for the rate of RecA assembly: From linear fits to the first ≈20 s of the assembly traces at F= 1.5 pN, we determine d θ/ d t ≈−0.14 turns s −1 and d z/ d t =−65 nm − s −1 for 0.5 μm radius beads ( Fig. 4b,c ) and d θ /d t ≈−0.024 turns s −1 and d z/ d t =−35 nm −1 s −1 for 1.4 μm radius beads ( Supplementary Fig. S15 ). With Δθ RecA =−44.7° per monomer and Δl RecA =0.53 nm per monomer determined from the overall geometry of the filament and Δl plec =40 nm per turns at F= 1.5 pN in similar buffer conditions [4] , [17] , we find d N RecA /d t= 13 monomer s −1 and 7.5 monomer s −1 for 0.5 and 1.4 μm beads, respectively, in good agreement with previous measurements on torsionally unconstrained DNA [21] , [22] . Analysis of the maximal number of plectonemes introduced at the end of the first fast RecA assembly phase suggests that RecA cannot assemble on plectonemic DNA. The initial phase terminates when the apparent tether extension reaches its minimum value ( ∼ 75 s as shown in red curve in inset to Fig. 4c ; see also inset to Supplementary Fig. S15 ), that is, when a maximal number of plectonemes have been formed. At this point, the change in tether length compared with bare DNA is Δz = N RecA × Δl RecA −ΔWr × Δl plec , where the first term corresponds to lengthening due to RecA binding and the second term to shortening due to plectoneme formation. Similarly, the change in tether rotation is Δθ=N RecA × Δθ RecA +ΔWr+ΔTw . Experimentally, we find Δz ≈1.5 μm and Δθ ≈−4 (the average of −7 turns for 0.5 μm radius beads and −1 turn for 1.4 μm radius beads; Supplementary Fig. S15 ). As RecA-covered DNA has a higher torsional stiffness than bare DNA [6] , we can approximate the change in twist accommodated by the tether by that of bare DNA of the same length before buckling at the same stretching force: ΔTw ≈23 turns. Combining these expressions for Δz and Δθ , we find ΔWr ≈−45 turns and N RecA ≈580 monomers at the end of the initial phase of fast filament assembly. The minimal extension of the tether during the assembly traces is ≈0.9 μm ( Supplementary Fig. S15 ), in agreement with the expected length of a filament of 580 RecA monomers assembled on DNA. This suggests that the initial phase of RecA assembly ends when the entire contour length of the DNA is partitioned between and RecA-covered stretches on the one hand and plectonemes on the other hand, consistent with previous observations, suggesting that RecA cannot assembly on plectonemic DNA [22] . In the second phase of RecA assembly, after the initial formation of plectonemes, both the tether length and unwinding angle, increase steadily. In this phase, bead rotation directly reports on drag-limited RecA filament assembly, evidenced by the fact that unwinding and lengthening proceeds and terminates concurrently ( Fig. 4b,c ). We have demonstrated that FOMT provide a straightforward way to measure the bias-free rotation of nucleic acid tethers, based on simple ( x,y ) tracking. We note that although it is possible to deduce changes in twist from length measurements in conventional MT [1] , [2] , [3] , [4] in the plectonemic regime, FOMT measurements are fundamentally different, as they directly measure changes in twist. In addition, in MT, one must perturb the system: conventional MT cannot measure at zero torque. Finally, as the rotating bead in FOMT permits the dissipation of torsional stress in the DNA molecule, it has the ability to measure unlimited changes in twist (for example, as a consequence of enzymatic activity), which is not possible in conventional MT. We note that the FOMT represents the ultimate limit of the recently introduced MTT [6] in which the stiffness of the magnetic torsional trap falls below that of the tether itself ( Fig. 3 ). Note that these two limits are readily interchangeable: FOMT measurements can, in principle, switch between torque application and twist measurement modes by attaching and detaching a small side magnet as it is used in the MTT. We can also compare the FOMT method with alternative approaches for (directly) tracking the rotation of nucleic acid tethers ( Supplementary Table S3 ). Compared with tethered particle motion assays [23] , [24] , the main advantage of the FOMT is the ability to apply calibrated and variable stretching forces. Previous studies using vertically aligned magnetic fields [25] , [26] , [27] are conceptually similar to FOMT, but have failed to demonstrate bias-free rotation ( Fig. 3 ) and have relied on fluorescence spectroscopy for the measurement of rotation. The MT–rotor bead assay [28] is most similar in performance to the FOMT. Unlike the FOMT, it uses distinct beads for force application and rotation detection, which may ultimately facilitate improved temporal resolution. However, this advantage of rotor-bead tracking comes at the expense of experimental complexity: disadvantages of this approach include the requirement of fluorescence spectroscopy for rotational measurement and the need for internal modification of the tether, limiting its applicability to studies of, for example, filament formation or RNA tethers. Finally, although a passive optical torque wrench [29] , [30] can, in principle, provide a similar assay, this technique has not yet been demonstrated for tethered particles, and achieving completely unconstrained rotation may prove challenging (zero torque application requires, in principle, infinitely fast polarization rotation). Furthermore, the requirements for an optical trap with sensitive polarization control and detection and for nanofabricated birefringent particles make the optical torque wrench experimentally challenging. In summary, compared with published techniques, FOMT achieves comparable or better specifications for angular resolution, temporal resolution and force range, and do so while significantly reducing experimental complexity. Leveraging an understanding of magnetic field, bead and tether geometry, FOMT provide a straightforward experimental strategy for measurements of changes in twist, without the need for fluorescence excitation or detection. The requirements for beads, tether constructs and position detection are identical to conventional MT. Any conventional MT can be converted to FOMT via the simple change of a low-cost magnet, requiring not a single change in the software, and hence put to immediate use in biophysical experiments. We envision that FOMT can be applied to a range of biological questions, for example, to monitor DNA-processing enzymes such as helicases and polymerases, to study DNA-binding small-molecule drugs and proteins and to explore properties of RNA and RNA–protein interactions. FOMT experimental configuration Tether construction and flow-cell assembly followed methods previously described in detail [6] , [31] . In brief, we used DNA tether constructs of 3.4, 7.9 or 20.6 kb length ligated at the ends to ≈600 bp DNA PCR fragments that were functionalized with multiple biotin and digoxigenin groups, respectively. Flow cells were made from glass microscope coverslips with parafilm spacers. The bottom surface was coated with nitrocellulose (0.1% wt/vol in amyl acetate) and flow cells were stored dry. Before measurements, 1.5 μm radius non-magnetic latex beads (Life Sciences) were unspecifically attached to the bottom surface by incubation in PBS (Sigma) buffer for 30 min to function as reference beads. Before addition of the DNA-linked magnetic beads, the bottom surface was functionalized by incubation with 100 μg ml −1 anti-digoxigenin (Roche) in PBS for 30 min, to provide for DNA attachment, and passivated by incubation for 30 min with 2 mg ml −1 bovine serum albumin (BSA) (Sigma). DNA molecules were first attached to streptavidin-coated superparamagnetic beads by incubation in PBS buffer for 30–60 min. Experiments used either 0.25–0.35 μm radius MagSense beads (MagSense), 0.5 μm radius MyOne beads (Invitrogen) or 1.4 μm radius M270 beads (Invitrogen). Finally, the DNA-tethered superparamagnetic beads were incubated in the flow cell for 30 min in PBS buffer to allow for DNA attachment to the anti-digoxigenin-coated surface. Forces were applied in the FOMT using a cylindrical permanent magnet with a centre hole formed by a stack of three magnets (R-06-02-02-G, Supermagnete) for a total thickness of 6 mm, with a diameter of 6 mm and a 2 mm diameter central hole. For measurements in the conventional MT configuration, we used pairs of 5×5×5 mm cubic magnets [8] (W-05-N50-G, Supermagnete). A linear stage (PI M-126.PD, Physik Instrumente) was used to change the distance of the magnet from the flow cell. Both the magnets and the flow cell were mounted on manual two-axis ( x,y )-micrometer stages, for alignment of the magnet centre and the magnetic beads, respectively. Some of the measurements used an additional computer-controlled ( x,y )-nanopositioning stage (733.2DD, Physik Instrumente) to move the flow cell over short distances with sub-micrometer precision and to use feedback to correct for drift. Beads were illuminated using a collimated LED and imaged using a ×100-oil immersion objective (Olympus ACH 100X; numerical aperture=1.25) connected to a CCD camera (Pulnix TM-6710CL). Buffer conditions For experiments with bare DNA, we used PBS buffer (137 mM NaCl, 2.7 mM KCl, 10 mM phosphate buffer, pH 7.4; Sigma) supplemented with 100 μg ml −1 BSA, 0.1% Tween and 5 mM sodium azide (PBS+). RecA experiments were performed in 20 mM 2-(N-morpholino)ethanesulfonic acid buffer (Sigma), pH 6.2, with 1 mM MgCl 2 (Sigma), 50 mM NaCl (Sigma), 1 mM dithiothreitol (Sigma) and 0.1 mM ATP-γS (Roche Diagnostics). We used commercially available RecA stock (New England Biolabs) at a final concentration of 5 μM. DNA tether calibrations All beads selected for experiments were confirmed to be tethered to the flow cell surface by a single, torsionally constrained dsDNA molecule as follows. The torsional constraint of the tethers was confirmed by rotating beads to positive turns (that is, overwinding the DNA) at F= 1.5–3.0 pN, and observing tether shortening due to plectoneme formation. We confirmed that beads were tethered by a single dsDNA molecule by comparing the response of the tether upon under- and overwinding at a stretching force of F =1.5–3.0 pN. Single dsDNA tethers shorten upon overwinding due to plectoneme formation, but do not shorten upon underwinding at these forces due to DNA melting [1] , [32] . In contrast, beads tethered to the surface by multiple dsDNA molecules show a symmetric decrease in length upon under- and overwinding as the tethers braid around one another. Fiducial marker beads for angular tracking For some of the measurements ( Supplementary Figs S9 and S10 ), we attached smaller, non-magnetic beads to M270 superparamagnetic beads after tethering of the magnetic beads to the surface, to function as fiducial markers for tracking of the beads' rotation [6] . As fiducials, we used biotin-labeled 0.5 μm radius Fluosphere microspheres (Invitrogen). Incubation of the flow cell with 1,000-fold diluted Fluosphere beads in PBS+ buffer for 30–60 min leads to stochastic attachment of fiducial beads to tethered magnetic beads. Tracking of bead position and rotation angle We used two different strategies to track the position of both the DNA-tethered and reference beads. One approach was to analyse bead images in real time using the conventional tracking algorithm based on cross-correlation analysis of the CCD bead images to determine their x , y and z positions [1] , [31] , [33] . For some measurements ( Supplementary Figs S9 and S10 ), we used a novel tracking algorithm that determines both the x , y and z positions and the rotation angle from analysis of images where a smaller 0.5 μm radius marker bead provided an asymmetry of the bead image [6] . This novel angular tracker was used to analyse pre-recorded images offline. The angular tracking is based on cross-correlation analysis of radial sections of the CCD images [6] and achieves an accuracy of ∼ 0.1° (J.L., J.W.J.K., Maylon Rojer and N.H.D., manuscript submitted). Converting the bead's ( x,y ) position to polar coordinates For a quantitative analysis of the fluctuations on the circular annulus, we converted the ( x , y ) position of the bead's centre to polar coordinates ( r , θ ) as follows: from a time trace of ( x i , y i ) positions, where the index i denotes subsequent measurement points, we fitted the circle centre ( x 0 , y 0 ) and radius R circle ( Fig. 1 and Supplementary Figs S2 and S3 ) by minimizing where the sum runs over all data points. After fitting x 0 , y 0 and R circle , the polar coordinates ( r i , θ i ) are given by where care was taken to 'unwrap' the angle θ , that is, appropriate phase jumps of ±π were added. Angular fluctuations in a harmonic potential In this section, we derive a quantitative description of a particle undergoing rotational fluctuations in an angular trap. The equation of motion in the rotational degree of freedom θ(t) is an overdamped Langevin equation: where γ is the rotational friction coefficient, k θ is the rotational trap stiffness and τ therm ( t ) is a Langevin torque from random collisions of the particle with the solvent. As the collisions are uncorrelated on the time scale of our measurement, τ therm ( t ) ∼ δ( t ). θ 0 =〈 θ ( t )〉 is the equilibrium angle of the trap, with the angled brackets denoting the time average. For simplicity, we can choose our coordinate system such that θ 0 =0. We define the autocorrelation function R(τ) as: By definition, the autocorrelation for zero time is equal to the variance of the angle. By the equipartition theorem, the variance of the angle is equal to the Boltzmann constant times the absolute temperature, k B T , divided by the trap stiffness, yielding: For τ >0 the integral over τ therm (t) in the definition of R(τ) averages to zero as the Brownian fluctuations are uncorrelated and R(τ) satisfies: with the solution: where we have defined the characteristic timescale of the system as τ c =γ/k θ . We find that the temporal autocorrelation of experimentally obtained angular time traces are well described by the exponential decay function of equation (16) ( Fig. 3e ; Supplementary Fig. S14 g ). From the exponential fit, both the trap stiffness k θ and the characteristic time τ c (or alternatively k θ and γ ) can be obtained. Alternatively, we can consider the power spectral density S ( f ) of the fluctuations that can be fitted by a Lorentzian [34] , [35] : where f c is the characteristic frequency of the system, with 2πf c = ω c and ω c =1/ τ c ( Fig. 3f ; Supplementary Fig. S15c ). Rotational friction coefficient The friction coefficient obtained from the fits to the temporal autocorrelation or power spectral density data can be compared with the value calculated from the bead geometry. A sphere of radius R bead rotating about an axis at a radial distance of R circle from its centre at a distance D from the surface has a rotational friction coefficient of: where η is the viscosity of the fluid, η ≈10 −3 kg m −1 s −1 for aqueous buffer. The denominators in equation (18) are the Faxen's corrections [36] , [37] due to the proximity of a surface to order O(( R bead /D ) 3 ). In our experiments, the bead is typically at least a distance of R bead but less than 3–4 R bead from the surface. In this range, the surface effects are modest, but non-negligible. As a numerical example, we predict a friction coefficient of γ =1.6 pN.nm.s for a configuration with R bead =0.35 μm and R circle =0.23 μm from equation (18), which is close to the experimentally measured value of γ =1.8 pN.nm.s ( Fig. 3 ). Measurement time scales and measurement accuracy The accuracy with which the equilibrium position θ 0 and fluctuations σ θ 2 can be measured depends on the number of independent samples recorded for the angle. As angular fluctuations are slow with respect to our camera, the number of independent samples in a measurement of time t meas is N = t meas /τ c . For the 3.4-kb DNA tethers used to determine the effective torsional stiffness C(F) of dsDNA from equilibrium fluctuations ( Fig. 2d ), τ c ∼ 2.5–10 s for 0.25–0.35 μm radius MagSense beads ( Supplementary Fig. 14 ) and τ c ∼ 15–30 s for 0.5 μm radius MyOne beads ( Supplementary Fig. 15 ). For each experiment to determine C(F) , we recorded traces ≥30 τ c in length, corresponding to traces of hundreds to thousands of seconds, giving a relative sampling error N −1/2 ≤20%. We note that for longer DNA constructs and larger beads, the characteristic time scale increases rapidly, for example, we find τ c ∼ 1000 s for R bead =1.4 μm and 7.9 kb DNA and τ c <2,500 s for R bead =1.4 μm and 20.6 kb DNA. When examining dynamics, the temporal resolution achievable given the bead sizes and tether lengths used must be taken into account, a fact that may have been overlooked in previous studies of rotation under vertically aligned MT [27] . How to cite this article: Lipfert, J. et al . Freely orbiting magnetic tweezers to directly monitor changes in the twist of nucleic acids. Nat. Commun. 2:439 doi: 10.1038/ncomms1450 (2011).